Structural basis for LAR-RPTP/Slitrk complex-mediated synaptic adhesion Synaptic adhesion molecules orchestrate synaptogenesis. The presynaptic leukocyte common antigen-related receptor protein tyrosine phosphatases (LAR-RPTPs) regulate synapse development by interacting with postsynaptic Slit- and Trk-like family proteins (Slitrks), which harbour two extracellular leucine-rich repeats (LRR1 and LRR2). Here we identify the minimal regions of the LAR-RPTPs and Slitrks, LAR-RPTPs Ig1–3 and Slitrks LRR1, for their interaction and synaptogenic function. Subsequent crystallographic and structure-guided functional analyses reveal that the splicing inserts in LAR-RPTPs are key molecular determinants for Slitrk binding and synapse formation. Moreover, structural comparison of the two Slitrk1 LRRs reveal that unique properties on the concave surface of Slitrk1 LRR1 render its specific binding to LAR-RPTPs. Finally, we demonstrate that lateral interactions between adjacent trans -synaptic LAR-RPTPs/Slitrks complexes observed in crystal lattices are critical for Slitrk1-induced lateral assembly and synaptogenic activity. Thus, we propose a model in which Slitrks mediate synaptogenic functions through direct binding to LAR-RPTPs and the subsequent lateral assembly of LAR-RPTPs/Slitrks complexes. Neuronal communication occurs at specialized asymmetrical junctions termed synapses. Synaptogenesis, which is the formation of a fully functional synapse, proceeds via a series of neuronal process that include the initial axon–dendrite contact, synapse formation and synapse maturation. Synaptic adhesion molecules located in the pre- and postsynaptic membranes play key roles in synaptogenesis. Similar to other cellular adhesion molecules (for example, those in tight junctions and immunological synapses), synaptic adhesion molecules physically align two neuronal cells and orchestrate the necessary bidirectional neuronal signalling pathways by forming trans -synaptic adhesion complexes [1] . The leukocyte common antigen-related receptor protein tyrosine phosphatases (LAR-RPTPs), which are classified as type IIa RPTPs, have recently emerged as a major family of synaptic adhesion molecules that also play crucial roles in neurite outgrowth, axon guidance and central nervous system (CNS) regeneration [2] , [3] . The vertebrate LAR-RPTP family has three members, LAR, PTPδ and PTPσ; their extracellular regions contain three immunoglobulin-like (Ig) domains and four to eight fibronectin III (FNIII) repeats (determined by alternative splicing). In particular, multiple LAR-RPTP isoforms are generated by alternative splicing of four mini exons, termed MeA to MeD, that encode short peptides ( Fig. 1a ) [4] , [5] . The LAR-RPTPs have a single transmembrane domain followed by two intracellular phosphatase domains (a membrane-proximal catalytic domain called D1 and a membrane-distal non-catalytic domain called D2) where multiple intracellular adaptor proteins bind [6] . Recently, a growing number of postsynaptic adhesion molecules have been identified as adhesion partners of the LAR-RPTPs; these include NGL-3 (netrin-G ligand 3), TrkC (neurotrophin receptor tyrosine kinase C), IL-1RAcP (interleukin 1 receptor accessory protein), IL1RAPL1 (IL-1 receptor accessory protein-like 1) and the Slitrks (Slit- and Trk-like family proteins) [2] , [3] . Two alternative splicing sites within the Ig domain of the LAR-RPTPs (MeA and MeB) have received particular attention, because they modulate the interactions with various postsynaptic ligands, such as TrkC, IL-1RAcP and IL1RAPL1 (refs 7 , 8 , 9 ). 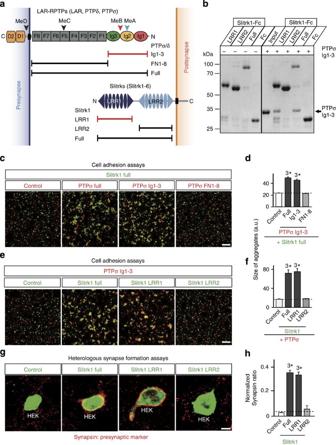Figure 1: Determination of minimal binding domains of PTPσ and Slitrk1. (a) Schematic domain structures of LAR-RPTPs and Slitrk family members. Abbreviations: Ig, Ig-like domain (Ig1, red; Ig2, yellow; and Ig3, green); F, fibronectin-like domain (grey); D1 and D2, phosphatase domains; N, N termini; C, C termini; LRR, leucine-rich repeat. The LRR1 and LRR2 domains of Slitrk1 are shown in dark blue and light blue, respectively. The relative positions of the MeA, MeB, MeC and MeD splice inserts are indicated by arrow head. Minimal binding domains are indicated with red lines. (b) Analysis of the interaction between PTPσ and Slitrk1 by pull-down assays. Recombinant Slitrk1 LRR1-Fc (~52 kDa), Slitrk1 LRR2-Fc (~52 kDa) or Slitrk1Full-Fc (~87 kDa) were immobilized using protein A-Sepharose, followed by incubation with PTPσ Ig1–3 (~33 kDa). Bound proteins were analysed by Coomassie Blue staining. (c–f) Representative images (c,e) and summary bar graphs (d,f) from our cell-adhesion assays. One group of L cells co-expressing DsRed and the indicated PTPσ variants was mixed with a second group of L cells co-expressing EGFP and indicated Slitrk1 variants. The dark grey bars are significantly different from the control, whereas the light grey bars are not significantly different atP<0.05. ‘n’ denotes the total number of cell aggregates from three independent experiments (200–1,000 aggregates from 5 to 9 cells); statistical significance indandfwas assessed using analysis of variance (ANOVA) with Tukey’s test (3*P<0.001). Error bars indandfrepresent s.d from three replicates. Scale bar, 100 μm. (g,h) Heterologous synapse-formation assays. HEK 293T cells transfected with EGFP alone (Control) or the indicated Slitrk1 variants were cocultured with hippocampal neurons and examined by double immunofluorescence using antibodies against GFP/HA (green) and synapsin (red). Representative images are shown (g), and the normalized synapse density is expressed as the ratio of synapsin staining to GFP/HA fluorescence (h). Results are expressed as means±s.d. (error bars) of three (n) independent experiments; statistical significance in (h) was assessed using ANOVA with Tukey’s test (3*P<0.001). Scale bar, 30 μm. Figure 1: Determination of minimal binding domains of PTPσ and Slitrk1. ( a ) Schematic domain structures of LAR-RPTPs and Slitrk family members. Abbreviations: Ig, Ig-like domain (Ig1, red; Ig2, yellow; and Ig3, green); F, fibronectin-like domain (grey); D1 and D2, phosphatase domains; N, N termini; C, C termini; LRR, leucine-rich repeat. The LRR1 and LRR2 domains of Slitrk1 are shown in dark blue and light blue, respectively. The relative positions of the MeA, MeB, MeC and MeD splice inserts are indicated by arrow head. Minimal binding domains are indicated with red lines. ( b ) Analysis of the interaction between PTPσ and Slitrk1 by pull-down assays. Recombinant Slitrk1 LRR1-Fc (~52 kDa), Slitrk1 LRR2-Fc (~52 kDa) or Slitrk1Full-Fc (~87 kDa) were immobilized using protein A-Sepharose, followed by incubation with PTPσ Ig1–3 (~33 kDa). Bound proteins were analysed by Coomassie Blue staining. ( c – f ) Representative images ( c , e ) and summary bar graphs ( d , f ) from our cell-adhesion assays. One group of L cells co-expressing DsRed and the indicated PTPσ variants was mixed with a second group of L cells co-expressing EGFP and indicated Slitrk1 variants. The dark grey bars are significantly different from the control, whereas the light grey bars are not significantly different at P <0.05. ‘ n ’ denotes the total number of cell aggregates from three independent experiments (200–1,000 aggregates from 5 to 9 cells); statistical significance in d and f was assessed using analysis of variance (ANOVA) with Tukey’s test ( 3 * P <0.001). Error bars in d and f represent s.d from three replicates. Scale bar, 100 μm. ( g , h ) Heterologous synapse-formation assays. HEK 293T cells transfected with EGFP alone (Control) or the indicated Slitrk1 variants were cocultured with hippocampal neurons and examined by double immunofluorescence using antibodies against GFP/HA (green) and synapsin (red). Representative images are shown ( g ), and the normalized synapse density is expressed as the ratio of synapsin staining to GFP/HA fluorescence ( h ). Results are expressed as means±s.d. (error bars) of three ( n ) independent experiments; statistical significance in ( h ) was assessed using ANOVA with Tukey’s test ( 3 * P <0.001). Scale bar, 30 μm. Full size image Among the LAR-RPTP ligands, the Slitrks were recently shown to induce presynaptic differentiation [10] , [11] . The six members of the Slitrk family (Slitrk1–6) are neuron-specific transmembrane proteins that localize at the postsynaptic membrane and exhibit domain structures similar to those of the classic axon guidance molecule, Slit [12] . All six Slitrks possess two leucine-rich repeat (LRR) domains in their extracellular regions; called LRR1 and LRR2, these domains are connected by a 70–90 amino acid loop. Each LRR domain has six LRR modules flanked by cysteine-rich regions at its amino terminus (LRRNT) and carboxy terminus (LRRCT) [12] . The Slitrk family members exhibit synaptogenic activities through their interactions with specific LAR-RPTP members [10] . Specifically, Slitrk1, Slitrk2, Slitrk4 and Slitrk5 promote excitatory synapse formation by interacting with PTPσ, whereas Slitrk3 enhances inhibitory synapse formation by interacting with PTPδ [10] . However, the lack of a high-resolution structure of the LAR-RPTP/Slitrk complex has limited our understanding of how these proteins act in synapse formation. Developing a greater understanding of the detailed molecular mechanisms underlying the functions of trans -synaptic adhesion pathways will be crucial for the future development of therapeutic strategies against a range of neurological disorders in which Slitrks and LAR-RPTPs have been implicated, including autism spectrum disorders, attention-deficit hyperactivity disorders, Tourette’s syndrome, trichotillomania and epilepsy [2] , [3] , [13] . Here we identified the minimal binding regions of the LAR-RPTPs and Slitrks, and determined the crystal structure of the resulting complex (PTPδ Ig1–3/Slitrk1 LRR1). We then performed an extensive functional analysis based on this complex structure and gained important insights into the molecular mechanism and the physiological significance of interactions between LAR-RPTPs and Slitrks in synaptogenesis. Our structural analysis of Slitrk1 LRR2 provided novel insights into how LAR-RPTPs specifically bind to Slitrk1 LRR1 but not Slitrk1 LRR2. Finally, from the crystal-packing lattices, we identified adjacent interactions between the convex surface of Slitrk LRR1 and the neighbouring PTPδ Ig1–3, and found that these lateral interactions are essential for Slitrk1-mediated surface cluster formation and presynaptic differentiation. These data suggest a model of the trans -adhesion complex wherein LAR-RPTPs and Slitrks coordinate synaptogenesis in a two-step process: direct binding of postsynaptic Slitrks to presynaptic LAR-RPTPs and subsequent lateral assembly in the formed complexes. Minimal domain identification for binding and synaptogenesis Our group and others recently demonstrated that LAR-RPTPs interact with Slitrks, and that this interaction contributes to regulating synapse formation and function [10] , [11] . To further characterize this interaction at the molecular level, we focused on PTPσ and Slitrk1, a trans -synaptic adhesion molecule pair that was shown to specifically promote excitatory synapse development [10] . We first generated three pDis-PTPσ constructs containing different extracellular domains: the full extracellular region (PTPσ Full), the three Ig domains alone (PTPσ Ig1–3) and the eight FNIII repeats alone (PTPσ FN1–8) ( Supplementary Table 1 ; see the architectures of LAR-RPTPs and Slitrks in Fig. 1a ). We then performed cell-adhesion assays with L cells expressing various PTPσ variants and the full extracellular region of Slitrk1 (Slitrk1 Full) ( Fig. 1c,d ). Consistent with our previous observation that LAR-RPTPs mediate the trans -interaction with Slitrks [10] , L cells expressing PTPσ full strongly aggregated with L cells expressing Slitrk1. The extent of aggregation among cells expressing PTPσ Ig1–3 was similar to that observed with PTPσ Full, indicating that PTPσ Ig1–3 is sufficient for Slitrk1 binding ( Fig. 1c,d ). PTPδ Ig1–3 also bound to Slitrk1 ( Supplementary Fig. 1 ). NGL-3 bound to the FNIII repeats but not to Ig1–3, which is consistent with a previous report that NGL-3 binds to the first two FNIII repeats of LAR-RPTPs [14] . The Slitrks contain two clusters of LRR modules, termed LRR1 and LRR2 (ref. 12 ) ( Fig. 1a ). We thus generated two additional pDis-Slitrk1 constructs containing LRR1 alone (Slitrk1 LRR1) or LRR2 alone (Slitrk1 LRR2), and performed cell-adhesion assays ( Fig. 1e,f ). L cells expressing Slitrk1 Full or Slitrk1 LRR1, but not Slitrk1 LRR2, strongly aggregated with L cells expressing PTPσ Ig1–3, indicating that Slitrk1 LRR1 mediates PTPσ binding ( Fig. 1e,f ). Consistent with the results from the cell-adhesion assays, recombinant PTPσ Ig1–3 or PTPδ Ig1–3 proteins specifically interacted with recombinant Slitrk1 Full or Slitrk1 LRR1, but not with Slitrk1 LRR2 ( Fig. 1b and Supplementary Fig. 1c,d ). In addition, the respective LRR1 domains of Slitrk2 and Slitrk3 also mediated interactions with PTPσ in cell-adhesion assays ( Supplementary Fig. 2a,b ). Collectively, these results indicate that Ig1–3 of the LAR-RPTPs and LRR1 of the Slitrks are sufficient for their mutual interactions. We next tested whether Slitrks LRR1 is sufficient to induce presynaptic differentiation. Heterologous synapse-formation assays showed that Slitrk1 LRR1, but not Slitrk1 LRR2, induced the clustering of the presynaptic vesicle protein, synapsin, in contacting axons of co-cultured neurons to an extent similar to that induced by Slitrk1 Full ( Fig. 1g,h ). Extending these heterologous synapse-formation assays to other Slitrks, we also found that the LRR1 domains of the other Slitrks were sufficient to induce presynaptic differentiation at a level similar to that triggered by their full-length extracellular counterparts ( Supplementary Fig. 2c,d ). Taken together, these results indicate that Slitrks orchestrate presynapse development through direct interactions with LAR-RPTPs, and that these interactions are mediated by their minimal binding regions, LAR-RPTPs Ig1–3 and Slitrk LRR1. Structure of minimal binding complex PTPδ Ig1–3/Slitrk1 LRR1 We initially sought to crystallize the physiological synaptic adhesion complex (PTPσ Ig1–3/Slitrk1 LRR1), but these attempts failed to yield complex crystals. Thus, to examine the atomic details of the interaction between LAR-RPTPs and Slitrks, we crystallized the PTPδ Ig1–3/Slitrk1 LRR1 complex and determined its structure at a resolution of 3.06 Å ( Table 1 ). Our analysis of the crystal structure of the PTPδ Ig1–3/Slitrk1 LRR1 complex revealed that PTPδ Ig1–3 binds to Slitrk1 LRR1 with a 1:1 stoichiometry, and the Ig2–3 domains of PTPδ contribute to this interaction ( Fig. 2a and Supplementary Fig. 3a ). Of the two splicing inserts of PTPδ Ig1–3 (MeA and MeB), only MeB was found to participate in the interaction with Slitrk1 (see below). Slitrk1 LRR1, which has the typical horseshoe shape of an LRR domain [15] , contains eight-stranded parallel β-sheets on the concave surface where PTPδ predominantly binds and variable loops on its convex surface. Table 1 Data collection and refinement statistics. 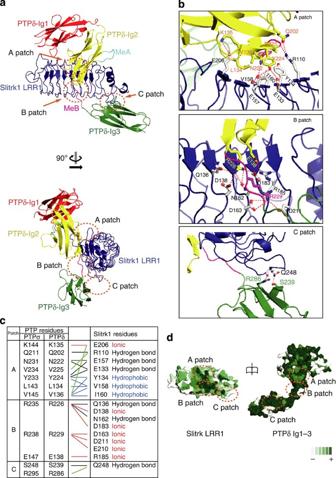Figure 2: Complex structure of the PTPδ Ig1–3/Slitrk1 LRR1. (a) Overview of the PTPδ Ig1–3/Slitrk1 LRR1 complex. The Ig1, Ig2 and Ig3 domains in PTPδ Ig1–3 and Slitrk1 LRR1 are coloured red, yellow, green and blue, respectively. The PTPδ splice inserts, MeA and MeB, are shown in cyan and magenta, respectively. The interacting regions are divided into the A, B and C patches as shown. (b) Close-up views of each binding interface. The residues involved in the interaction are displayed as sticks and labelled. Hydrogen and ionic bonds are indicated by dashed red lines. (c) Key amino acid residues involved in the interactions within the A, B and C patches. Residues of PTPδ and the corresponding residues of PTPσ are listed on the left, and the residues of Slitrk1 are listed on the right. Interactions between residue partners are indicated by red (ionic interaction), black (hydrogen bond), blue (hydrophobic interaction) and green (main-chain interaction) lines. (d) Sequence conservations were calculated by the Consurf server16and are presented on the surfaces of Slitrk1 LRR1 (left) and PTPδ Ig1–3 (right). Dark green represents higher conservation. The structures are shown in the open-book view and the orientation of the surface view of LRR1 is identical to that ina(top). Full size table Figure 2: Complex structure of the PTPδ Ig1–3/Slitrk1 LRR1. ( a ) Overview of the PTPδ Ig1–3/Slitrk1 LRR1 complex. The Ig1, Ig2 and Ig3 domains in PTPδ Ig1–3 and Slitrk1 LRR1 are coloured red, yellow, green and blue, respectively. The PTPδ splice inserts, MeA and MeB, are shown in cyan and magenta, respectively. The interacting regions are divided into the A, B and C patches as shown. ( b ) Close-up views of each binding interface. The residues involved in the interaction are displayed as sticks and labelled. Hydrogen and ionic bonds are indicated by dashed red lines. ( c ) Key amino acid residues involved in the interactions within the A, B and C patches. Residues of PTPδ and the corresponding residues of PTPσ are listed on the left, and the residues of Slitrk1 are listed on the right. Interactions between residue partners are indicated by red (ionic interaction), black (hydrogen bond), blue (hydrophobic interaction) and green (main-chain interaction) lines. ( d ) Sequence conservations were calculated by the Consurf server [16] and are presented on the surfaces of Slitrk1 LRR1 (left) and PTPδ Ig1–3 (right). Dark green represents higher conservation. The structures are shown in the open-book view and the orientation of the surface view of LRR1 is identical to that in a (top). Full size image The binding interface could be divided into three distinct regions termed the A, B and C patches ( Fig. 2a ). Their buried surface areas were 741, 535 and 497 Å 2 , respectively, and all residues involved in the interactions of each patch are presented in Fig. 2b,c . The A patch is formed by the A′-G/G′-F-C β-sheet of the PTPδ Ig2 domain and the upper parts of the β3~β5 strand on the concave surface of Slitrk1 LRR1. In the A patch, multiple electrostatic interactions are mediated by residues of the PTPδ Ig2 domain (K135, Q202, N222 and Y224) and Slitrk1 LRR1 (R110, E133, E157 and E206), which surround the network of hydrophobic core interactions ( Fig. 2b,c ). The B patch interaction, which occurs between the Ig2-MeB splice inserts of PTPδ and the lower parts of the β4~β6 strand on the concave surface of Slitrk1 LRR1, is mainly mediated by ionic interactions and hydrogen bonds. In particular, two positively charged arginine residues of PTPδ (R226 in Ig2 βG′ and R229 in MeB) bind respectively to two negatively charged arginine pockets in Slitrk1 LRR1 (Arg pockets 1 and 2). Arg pocket 1 is composed of Q136, D138, N162 and D183, while Arg pocket 2 is composed of D163, G186, E210 and D211 ( Fig. 2b and Supplementary Fig. 3b ). The C patch contains two hydrogen bonds, S239 and R286, in the Ig3 domain of PTPδ, which bind the side-chain amide and backbone carbonyl of Q248, respectively, in the LRRCT of Slitrk1 LRR1. The C patch interaction probably contributes to holding the PTPδ Ig3 domain in a rigid arrangement, preventing it from swinging around on the flexible loop located between Ig2 and Ig3 of PTPδ. A conservation analysis was performed on the sequences listed in Supplementary Table 2 , using the Consurf server [16] . It showed that in the A, B and C patches, the key residues involved in the interaction are highly conserved with the exception of E157 and Q248 of Slitrk1 ( Fig. 2d and Supplementary Fig. 4 ). Critical residues for presynaptic differentiation The overall structures of Ig1–2 of PTPδ and PTPσ are almost identical [17] . Our in vitro biochemical and cell biological experiments also showed that both PTPδ Ig1–3 and PTPσ Ig1–3 bind equally well to Slitrk1 LRR1 ( Fig. 1 and Supplementary Figs 1 and 2 ). Moreover, additional analyses revealed that the PTPδ residues involved in the interaction with Slitrk1 were exactly identical to the corresponding critical residues of PTPσ ( Supplementary Fig. 4 ). Thus, we hypothesized that the mode through which PTPσ Ig1–3 binds to Slitrk1 LRR1 should be analogous to that of PTPδ Ig1–3. On the basis of this assumption, and guided by the structural information obtained from the PTPδ Ig1–3/Slitrk1 LRR1 complex, we designed a series of PTPσ and Slitrk1 mutations that we predicted to abolish mutual binding or alter the binding interfaces, presumably changing their respective binding properties ( Fig. 3a ). 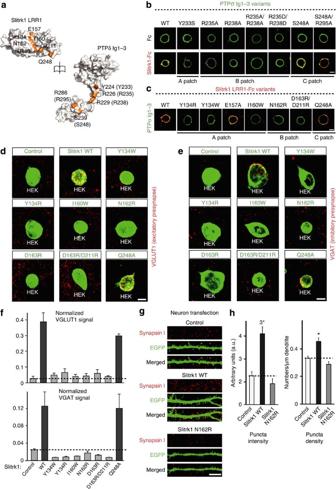Figure 3: Critical residues for PTPσ/Slitrk1 binding and synaptogenic activity. (a) An open-book view showing the interacting interfaces of the PTPδ Ig1–3/Slitrk1 LRR1 complex. The orientations of PTPδ and Slitrk1 are identical to those inFig. 2d. The amino acid residues mutated for our functional analyses are labelled and shown in orange; the residue numbers of PTPσ are shown in parentheses. (b) Cell surface binding assays performed with HEK293T cells expressing PTPσ Ig1–3 WT or its various mutants. Cells were analysed by immunofluorescence imaging for Slitrk1 LRR1-Fc (red) and HA-tagged PTPσ Ig1–3 (green). Scale bar, 20 μm. (c) Cell surface binding assays were performed as described inb, except that the HEK293T cells expressing PTPσ Ig1–3 WT were incubated with Fc or the indicated Slitrk1 LRR1-Fc variants. Scale bar, 20 μm. (d–f) Representative immunofluorescence images (d,e) and summary bar graphs (f) for our heterologous synapse-formation assays. Hippocampal cultured neurons were cocultured with HEK293T cells expressing mVenus alone (Control), Slitrk1 WT fused with mVenus (Slitrk1 WT), or various Slitrk1 mutants fused with mVenus (Y134R, Y134W, E157A, I160W, N162R, D163R/D211R or Q248A) and stained with antibodies against EGFP (green) and excitatory (VGLUT1;d) or inhibitory (VGAT;e) presynaptic markers (red). Results are expressed as means±s.d. (error bars) of three (n) independent experiments; statistical significance infwas assessed using analysis of variance (ANOVA) with Tukey’s test. Darker grey bars are significantly different from control (3*P<0.001). (g) Rat hippocampal neurons were transfected with GFP (Control), Slitrk1 WT or Slitrk N162R, and stained for the synaptic maker, synapsin (red) and EGFP (green). Scale bar, 5 μm. (h) Quantification of the synaptic density shown ing. Results are expressed as means±s.d. (error bars) of three (n) independent experiments; statistical significance inhwas assessed using ANOVA with Tukey’s test (3*P<0.001). Figure 3: Critical residues for PTPσ/Slitrk1 binding and synaptogenic activity. ( a ) An open-book view showing the interacting interfaces of the PTPδ Ig1–3/Slitrk1 LRR1 complex. The orientations of PTPδ and Slitrk1 are identical to those in Fig. 2d . The amino acid residues mutated for our functional analyses are labelled and shown in orange; the residue numbers of PTPσ are shown in parentheses. ( b ) Cell surface binding assays performed with HEK293T cells expressing PTPσ Ig1–3 WT or its various mutants. Cells were analysed by immunofluorescence imaging for Slitrk1 LRR1-Fc (red) and HA-tagged PTPσ Ig1–3 (green). Scale bar, 20 μm. ( c ) Cell surface binding assays were performed as described in b , except that the HEK293T cells expressing PTPσ Ig1–3 WT were incubated with Fc or the indicated Slitrk1 LRR1-Fc variants. Scale bar, 20 μm. ( d – f ) Representative immunofluorescence images ( d , e ) and summary bar graphs ( f ) for our heterologous synapse-formation assays. Hippocampal cultured neurons were cocultured with HEK293T cells expressing mVenus alone (Control), Slitrk1 WT fused with mVenus (Slitrk1 WT), or various Slitrk1 mutants fused with mVenus (Y134R, Y134W, E157A, I160W, N162R, D163R/D211R or Q248A) and stained with antibodies against EGFP (green) and excitatory (VGLUT1; d ) or inhibitory (VGAT; e ) presynaptic markers (red). Results are expressed as means±s.d. (error bars) of three ( n ) independent experiments; statistical significance in f was assessed using analysis of variance (ANOVA) with Tukey’s test. Darker grey bars are significantly different from control ( 3 * P <0.001). ( g ) Rat hippocampal neurons were transfected with GFP (Control), Slitrk1 WT or Slitrk N162R, and stained for the synaptic maker, synapsin (red) and EGFP (green). Scale bar, 5 μm. ( h ) Quantification of the synaptic density shown in g . Results are expressed as means±s.d. (error bars) of three ( n ) independent experiments; statistical significance in h was assessed using ANOVA with Tukey’s test ( 3 * P <0.001). Full size image To examine the significance of each interaction patch in PTPσ, we introduced the following specific point mutations in pDis-PTPσ Ig1–3 ( Supplementary Table 3 ): Y233S, which was intended to disrupt hydrophobic interactions in the A patch; R235A, R238A and R235D/R238D, which were intended to disrupt complementary charge interactions in the B patch; and S248A and R295A, which were intended to disrupt the two hydrogen bonds in the C patch. We expressed PTPσ Ig1–3 wild-type (WT) and each PTPσ Ig1–3 mutant on the surface of HEK293T cells and used cell surface-binding assays to measure the binding of recombinant Slitrk1-Fc WT proteins to these PTPσ variants ( Fig. 3b ). All of the mutants were defective for Slitrk1 binding, except for two (PTPσ Ig1–3 S248A and PTPσ Ig1–3 S248A/R295A) (see Supplementary Fig. 5e for binding-affinity data). We obtained consistent results from additional cell-adhesion assays ( Supplementary Fig. 5a,c ). We also designed a series of Slitrk1 mutants to disrupt the binding to PTPσ Ig1–3 and generated recombinant Slitrk1-Fc proteins (WT and various point mutants in Slitrk1; Fig. 3c ). We then performed cell surface-binding assays with HEK293T cells expressing PTPσ Ig1–3 WT. We found that all of the tested mutants abolished the binding of PTPσ Ig1–3, with the exception of two point mutants in Slitrk1: E157A in the A patch and Q248A in the C patch ( Fig. 3c ). Similar results were obtained from cell-adhesion assays performed with L cells expressing PTPσ Ig1–3 and the Slitrk1 variants ( Supplementary Fig. 5b,d ; see also Supplementary Fig. 5e for binding-affinity data). These findings collectively suggest that highly conserved residues in the A and B patches are required for this interaction. Slitrks have been shown to potently induce presynaptic differentiation in heterologous synapse-formation assays [10] , [11] . Intriguingly, Slitrk1 triggers presynaptic differentiation at both excitatory and inhibitory synapses and requires distinct LAR-RPTP isoforms for the specification of distinct synapse types [10] . Thus, we examined whether Slitrk1 point mutants defective in LAR-RPTP binding activity could induce presynaptic differentiation in heterologous synapse-formation assays. The expression level of each Slitrk1 point mutant (constructed in a pCMV5-Slitrk1-mVenus backbone) was quantified based on the mVenus moiety and the amount of synapse formation by transfected HEK293T cells was assessed using indirect immunofluorescent detection of the presynaptic marker proteins, VGLUT1 (vesicular glutamate transporter 1, an excitatory presynaptic marker) and VGAT (vesicular GABA transporter, an inhibitory presynaptic marker) ( Fig. 3d–f ). Consistent with our cell surface-binding and cell-adhesion assays, all Slitrk1 mutants that lacked PTPσ binding were unable to induce synapse formation ( Fig. 3d–f ). Biotinylation assays and indirect immunofluorescence assays showed that all of the Slitrk1 mutants were well expressed at the cell surface, except for Slitrk1-I160W and Slitrk1-D163R/D211R ( Supplementary Fig. 6a,b ). To overcome the poor surface transport of some Slitrk1 mutants, we expressed the Slitrk1 variants (pDis-HA-Slitrk1) at the cell surface of HEK293T cells and conducted heterologous synapse-formation assays. All of the Slitrk1 mutants failed to induce synapse formation, with the exception of Slitrk1-Q248A ( Supplementary Fig. 6c,d ). Next, we transfected rat hippocampal neurons with vectors encoding enhance green fluorescence protein (EGFP) alone (Control), mVenus-fused WT and EGFP (Slitrk1 WT), or mVenus-fused Slitrk1 N162R and EGFP (Slitrk1 N162R), and immunostained the neurons for the synaptic marker, synapsin. We found that overexpression of Slitrk1 WT significantly increased the fluorescence intensity and linear density of the synapsin puncta on dendrites of transfected neurons, whereas overexpression of the Slitrk1 N162R mutant did not ( Fig. 3g,h ). These results suggest that Slitrk1 uses the same binding interfaces in the A and B patches to induce presynaptic differentiation at both excitatory and inhibitory synapses, and further indicate that Slitrk1 promotes excitatory synapse development by directly binding to PTPσ in cultured hippocampal neurons. Splicing insert MeB modulates LAR-RPTPs/Slitrk interaction The alternative splice variants in the Ig domains of the LAR-RPTPs selectively modulate their binding affinity to multiple postsynaptic partners, including TrkC, IL-1RAcP and IL1RAPL1 (refs 7 , 8 , 9 ). The crystal structure of the PTPδ Ig1–3/Slitrk1 LRR1 complex and our mutant analyses clearly demonstrated that an arginine residue within MeB critically determines the interaction between PTPσ and Slitrk1 LRR1 ( Figs 2 and 3 ). Structural comparisons of PTPδ Ig1–3 in the presence (current study) and absence [17] of MeB (PDB ID: 2YD9) revealed that the shortened linker between Ig2 and Ig3 of PTPσ Ig1–3 lacking MeB (PTPσ Ig1–3 MeA+, MeB−) introduces a conflict between the Ig3 domain and Slitrk1 LRR1, even though the overall architecture of the individual Ig domains and the V-shape of the rigid Ig1–Ig2 unit are well preserved ( Fig. 4a and Supplementary Fig. 7 ). Interestingly, the position of Ig3 in PTPδ Ig1–3 (MeA+, MeB+) was rotated about 62° around V225, which is the last residue in the βG’ sheet of PTPδ Ig2 ( Fig. 4a , left). As shown in Fig. 3 , however, the C patch interaction is not critical for the binding of Slitrk1 to LAR-RPTPs or the mediation of presynaptic differentiation; thus, the significance of this rotational shift is not clear. Our structural analysis indicated that MeB contributes to the binding of LAR-RPTPs to Slitrks by: (1) fitting PTPδ R229 (PTPσ R238) directly into Arg pocket 2 on Slitrk1 LRR1; (2) stabilizing the flexible PTPδ R226 (PTPσ R235) into Arg pocket 1 on Slitrk1 LRR1; and (3) increasing the length of the linker between Ig2 and Ig3 (Ig2–Ig3 linker), thereby relieving potential steric hindrance between LAR-RPTPs and Slitrks ( Fig. 4a , right). Next, we tested whether the interactions between PTPσ and Slitrk1 LRR1 are mainly regulated by the residues of MeB themselves or by the longer Ig2–Ig3 linker in PTPσ Ig1–3 (MeA+, MeB+). To mimic the short Ig2–Ig3 linker of PTPσ Ig1–3 (MeA+, MeB−), we deleted the three residues (EVR) after R238 in PTPσ Ig1–3 (MeA+, MeB+) without changing the residues in MeB (blue box in Supplementary Fig. 4 ) to create PTPσ-ΔEVR. Intriguingly, cell surface binding assays using HEK293T cells expressing various PTPσ Ig1–3 splice variants and PTPσ-ΔEVR showed that recombinant Slitrk1-Fc bound to PTPσ-ΔEVR and a subset of PTPσ splice variants that contain MeB (that is, PTPσ Ig1–3 (MeA−, MeB+) and PTPσ Ig1–3 (MeA+, MeB+); Fig. 4b ). These results are consistent with those obtained from our cell-adhesion assays ( Fig. 4c ), suggesting that the residues of the splicing insert, MeB, are more crucial than the length of the Ig2–Ig3 linker for the interaction with Slitrk1. To test this idea, we carried out lentiviral knockdown (KD) of PTPσ and rescue experiments. Lentiviral-mediated PTPσ KD in cultured hippocampal neurons abolished the ability of Slitrk1 to cluster VGLUT1, consistent with our previous report (Yim et al . [10] ; Supplementary Fig. 8e–g ). Re-expression of full-length PTPσ (MeA−, MeB+), but not full-length PTPσ (MeA−, MeB−), completely restored the synaptogenic activity of Slitrk1, consistent with our binding data (see Fig. 4 ). Moreover, the presence of MeB in PTPδ and LAR was also critical for Slitrk1 binding ( Supplementary Fig. 8a–d ). 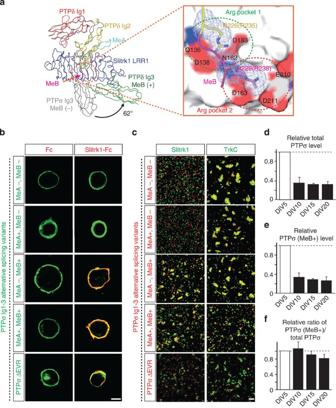Figure 4: Splicing inserts MeB of LAR-RPTPs modulates Slitrks binding. (a) Structural comparison of LAR-RPTPs in the presence and absence of MeB splicing inserts (left) and close-up view of arginine pockets on Slitrk1 LRR1 (right). The colour coding of PTPδ Ig1–3 (MeA+, MeB+) is as described inFig. 2a, and the structure of PTPσ Ig1–3 lacking MeA and MeB (2YD9) is shown in grey. Compared with the Ig3 domain of PTPσ Ig1–3 (MeA-, MeB-), the Ig3 domain in the PTPδ Ig1–3 (MeA+, MeB+) was rotated by 62° around V225, which is the last residue of the second Ig2 domain in PTPδ. (b) HEK293T cells expressing the indicated splice variants of PTPσ Ig1–3 were incubated with Slitrk1 LRR-Fc and analysed by immunofluorescence for Slitrk1 LRR1-Fc (red) and HA-tagged PTPσ Ig1–3 variants (green). Scale bar, 20 μm. (c) Representative images from our cell-adhesion assays. One group of L cells co-expressing DsRed and the indicated PTPσ variants was mixed with a second group of L cells co-expressing EGFP and Slitrk1 (Slitrk1) or TrkC (TrkC). Scale bar, 100 μm (applies to all images). TrkC bound to all splice variants of PTPσ, whereas Slitrk1 specifically interacted with PTPσ variants containing the splicing insert, MeB. (d–f) Bar graphs representing quantitative real-time RT–PCR results obtained from hippocampal neurons at the indicated time points, measuring relative mRNA levels of total PTPσ (d), the relative mRNA levels of PTPσ variants containing MeB (e) and the proportion of PTPσ variants containing MeB (f). The data were normalized with respect to the values obtained at DIV5 (defined as 1.0). Results are expressed as means±s.d. (error bars) of three (n) independent experiments; statistical significance (d–f) was assessed using analysis of variance with Tukey’s test. Black bars are significantly different compared with DIV5 groups (3*P<0.001). Figure 4: Splicing inserts MeB of LAR-RPTPs modulates Slitrks binding. ( a ) Structural comparison of LAR-RPTPs in the presence and absence of MeB splicing inserts (left) and close-up view of arginine pockets on Slitrk1 LRR1 (right). The colour coding of PTPδ Ig1–3 (MeA+, MeB+) is as described in Fig. 2a , and the structure of PTPσ Ig1–3 lacking MeA and MeB (2YD9) is shown in grey. Compared with the Ig3 domain of PTPσ Ig1–3 (MeA-, MeB-), the Ig3 domain in the PTPδ Ig1–3 (MeA+, MeB+) was rotated by 62° around V225, which is the last residue of the second Ig2 domain in PTPδ. ( b ) HEK293T cells expressing the indicated splice variants of PTPσ Ig1–3 were incubated with Slitrk1 LRR-Fc and analysed by immunofluorescence for Slitrk1 LRR1-Fc (red) and HA-tagged PTPσ Ig1–3 variants (green). Scale bar, 20 μm. ( c ) Representative images from our cell-adhesion assays. One group of L cells co-expressing DsRed and the indicated PTPσ variants was mixed with a second group of L cells co-expressing EGFP and Slitrk1 (Slitrk1) or TrkC (TrkC). Scale bar, 100 μm (applies to all images). TrkC bound to all splice variants of PTPσ, whereas Slitrk1 specifically interacted with PTPσ variants containing the splicing insert, MeB. ( d – f ) Bar graphs representing quantitative real-time RT–PCR results obtained from hippocampal neurons at the indicated time points, measuring relative mRNA levels of total PTPσ ( d ), the relative mRNA levels of PTPσ variants containing MeB ( e ) and the proportion of PTPσ variants containing MeB ( f ). The data were normalized with respect to the values obtained at DIV5 (defined as 1.0). Results are expressed as means±s.d. (error bars) of three ( n ) independent experiments; statistical significance ( d – f ) was assessed using analysis of variance with Tukey’s test. Black bars are significantly different compared with DIV5 groups ( 3 * P <0.001). Full size image In the case of neurexins, which are highly polymorphic owing to extensive alternative splicing [18] , the alternative splicing events are frequently modulated by synaptic activity [19] . To examine the temporal regulation of alternative splicing in PTPσ and PTPδ during neuronal development, we used quantitative reverse transcription–PCR (qRT–PCR) to monitor the expression levels of the PTPσ/δ messenger RNA in cultured rat hippocampal neurons. The mRNA levels of total PTPσ/δ and the splicing isoform PTPσ/δ (MeB+), both sharply decreased in cultured hippocampal neurons between DIV5 (days in vitro ) and DIV10, and remained consistent thereafter ( Fig. 4d,e and Supplementary Fig. 8h,i ). Moreover, the proportion of MeB-containing PTPσ/δ remained unchanged during postnatal brain development ( Fig. 4f and Supplementary Fig. 8j ). These data suggest that PTPσ/δ (MeB+) might be a dominant splice variant of PTP σ/δ in the developing rat hippocampus, and that the trans -synaptic complex containing LAR-RPTPs and Slitrks might be important for initial synapse formation, rather than late-stage synapse maturation. Structural differences between Slitrk1 LRR1 and LRR2 To examine the structural basis underlying the selective binding of LAR-RPTPs to Slitrk LRR1, we performed a crystallographic analysis of Slitrk1 LRR2 ( Fig. 5 , Supplementary Fig. 9d and Table 1 ). As a model template for molecular replacement, we used the variable lymphocyte receptor A, VLRA.R2.1, which has an LRRNT, six LRR motifs and an LRRCT (PDB ID: 3M18) [20] . The elution profile obtained from size-exclusion chromatography showed that Slitrk1 LRR2 existed in the monomeric form in the solution. However, the asymmetrical unit of the Slitrk1 LRR2 crystal contained two identical (Cα root mean squared deviation: 0.61 Å) monomers arranged as a face-to-face dimer via their concave surfaces. The overall structure of Slitrk1 LRR2 comprises nine β-strands on the concave face and secondary-structure-free loops on the convex surface. Slitrk1 LRR1 and LRR2 exhibit high structural homology, with a Cα root mean squared deviation of 1.035 Å. The loop connecting the anti-parallel strand in the LRRNT of the Slitrk1 LRR2 domain was slightly different from that in Slitrk1 LRR1 ( Fig. 5a,c ). 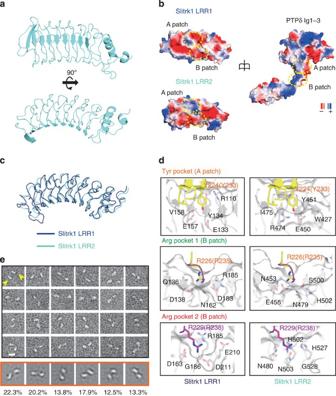Figure 5: Structural comparison of Slitrk1 LRR1 and LRR2 domains. (a) Cartoon representation of the structure of Slitrk1 LRR2. The two views are rotated by 90° along the horizontal axis. (b) Electrostatic potential of Slitrk1 LRR1, LRR2 and PTPδ Ig1–3, as calculated by the Poisson–Boltzmann equation in PyMOL. The structures are shown as open-book views and surface representations, with colour maps reflecting electrostatic properties (blue, positively charged; red, negatively charged). The interfaces involved in electrostatic interactions are highlighted by dashed circles. (c) Superposition of Slitrk1 LRR1 (dark blue) and Slitrk1 LRR2 (light blue), both depicted as ribbon diagrams. (d) The binding pockets for Y224 in PTPδ (Y233 for PTPσ; top), R226 in PTPδ (R235 for PTPσ; middle) and R229 in PTPδ (R238 for PTPσ; bottom) within the A and B patches of LRR1 are shown as sticks and surfaces in the left panel. Their corresponding positions in LRR2 are shown in the right panel. The PTPδ residues that dock into the Slitrk1 pockets are represented as coloured sticks (yellow for the Ig2 domain and magenta for the splicing insert, MeB). The residue numbers of PTPσ are shown in parentheses. (e) Representative negative-stained electron microscopy images of Slitrk1 Full ectodomain (yellow arrows indicate the horseshoe-shaped LRR domains). The typical horseshoe-shaped structures and the randomness of the relative positions of each LRR domain can be observed from the two-dimensional class averages displayed in the orange box. Among 1,403 particles, the percentile of particle numbers of each class are shown below each class average. Scale bar, 10 nm. Figure 5: Structural comparison of Slitrk1 LRR1 and LRR2 domains. ( a ) Cartoon representation of the structure of Slitrk1 LRR2. The two views are rotated by 90° along the horizontal axis. ( b ) Electrostatic potential of Slitrk1 LRR1, LRR2 and PTPδ Ig1–3, as calculated by the Poisson–Boltzmann equation in PyMOL. The structures are shown as open-book views and surface representations, with colour maps reflecting electrostatic properties (blue, positively charged; red, negatively charged). The interfaces involved in electrostatic interactions are highlighted by dashed circles. ( c ) Superposition of Slitrk1 LRR1 (dark blue) and Slitrk1 LRR2 (light blue), both depicted as ribbon diagrams. ( d ) The binding pockets for Y224 in PTPδ (Y233 for PTPσ; top), R226 in PTPδ (R235 for PTPσ; middle) and R229 in PTPδ (R238 for PTPσ; bottom) within the A and B patches of LRR1 are shown as sticks and surfaces in the left panel. Their corresponding positions in LRR2 are shown in the right panel. The PTPδ residues that dock into the Slitrk1 pockets are represented as coloured sticks (yellow for the Ig2 domain and magenta for the splicing insert, MeB). The residue numbers of PTPσ are shown in parentheses. ( e ) Representative negative-stained electron microscopy images of Slitrk1 Full ectodomain (yellow arrows indicate the horseshoe-shaped LRR domains). The typical horseshoe-shaped structures and the randomness of the relative positions of each LRR domain can be observed from the two-dimensional class averages displayed in the orange box. Among 1,403 particles, the percentile of particle numbers of each class are shown below each class average. Scale bar, 10 nm. Full size image Sequence conservation analysis showed that the binding interfaces of Slitrk1 LRR1 are highly conserved, whereas the corresponding areas in Slitrk1 LRR2 are more variable ( Supplementary Fig. 9a ). In addition, the charge distribution of Slitrk1 LRR1 is precisely complementary to that of PTPδ Ig1–3 over the binding interfaces, whereas the charges of Slitrk1 LRR2, particularly in the area that corresponds to the A patch of Slitrk1 LRR1, conflict with those of PTPδ Ig1–3 ( Fig. 5b ). We also examined the electrostatic properties of other Slitrks, using model structures generated by comparative homology modelling [21] , and found that similar charge conflicts were present on the concave surfaces of the LRR2 domains ( Supplementary Fig. 9b ). The conserved residues, Y233 (A patch), R235 (B patch) and R238 (B patch) in PTPσ Ig1–3 (corresponding residues for PTPδ Ig1–3: Y224, R226 and R229, respectively) fit into three distinct pockets on the concave surface of Slitrk1 LRR1: the tyrosine (Tyr) pocket in the A patch and arginine (Arg) pockets 1 and 2 in the B patch, respectively ( Fig. 5d , left panels). The Tyr pocket is formed by R110, E133, Y134, E157 and V158 of Slitrk1; Arg pocket 1 is formed by Q136, D138, N162, D183 and R185 of Slitrk1; and Arg pocket 2 is formed by D163, R185, G186, E210 and D211 of Slitrk1. A structural comparison of the Slitrk1 LRR1-binding pockets with the corresponding areas in Slitrk1 LRR2 showed that the conserved D138, V158 and G186 residues that contribute to formation of the shallow pockets in Slitrk1 LRR1 are replaced by amino acid residues with longer side chains (E455, I475 and N503) in Slitrk1 LRR2, resulting in occlusion of the binding pockets. These structural differences in the binding pockets could prevent LAR-RPTPs from binding to Slitrk1 LRR2 ( Fig. 5d , right panels). Taken together, these results suggest that unique properties on the concave surface of Slitrk1 LRR1, such as the binding pockets and complementary charge distributions, are key determinants for the specific interaction of LAR-RPTPs with Slitrk LRR1. What, then, is the role of Slitrk LRR2? Among the many LRR-containing neuronal proteins, the axon guidance molecule, Slit, has four consecutive LRR domains in its extracellular region, each of which executes a different role; for example, the D2 domain is responsible for the interaction with the ligand protein Roundabout (Robo), while the D4 domain is responsible for Slit dimerization [22] . Thus, we examined whether the LRR2 domain induces dimerization of Slitrks in a manner similar to that of the Slit D4 domain, or if it could regulate LAR-RPTPs/Slitrks complex formation by masking the LAR-RPTPs-binding surface on Slitrk LRR1. Negatively stained electron microscopic analysis of recombinant Slitrk1 Full revealed that the relative positions of Slitrk1 LRR1 and LRR2 are random, and the linker region between Slitrk1 LRR1 and LRR2 is highly flexible ( Fig. 5e and Supplementary Fig. 10 ). Individual Slitrk1 LRR1 and LRR2 domains adopted curved conformations resembling horseshoes, consistent with our crystal structures (marked with yellow arrows in Fig. 5e ). However, the LRR domains of Slitrk1 could not be distinguished from each other in the low-resolution electron microscopic image, owing to their structural similarity. In addition, we did not observe intermolecular interactions for dimerization, nor did we detect intramolecular interactions between LRR1 and LRR2 of Slitrk1. Based on these results, we speculate that Slitrk LRR2 might perform other functions, such as binding to unidentified binding protein(s). Lateral clustering of PTPσ/Slitrk1 complexes for synaptogenesis Previously, a hypothetical model was postulated wherein the higher-order assemblies of the neurexin/neuroligin synaptic adhesion complex are required for the presynaptic differentiation activity of neuroligins [23] , [24] . In addition, functional forward and reverse Eph/Ephrin synaptic adhesion signalling requires formation of higher-order clusters, initiated by initial contact between them in trans , followed by formation of larger signalling clusters and ultimately leading to lateral recruitment of additional Eph clusters [25] , [26] . Similar adhesion-promoted lateral clustering has been reported for cadherins [27] . Although an asymmetrical unit of the PTPδ Ig1–3/Slitrk1 LRR1 complex crystal was found to contain only one molecule of this complex, two discrete packing interactions along the two-fold screw symmetrical axis were observed between adjacent PTPδ Ig1–3/Slitrk1 complexes in the crystal-packing lattice ( Fig. 6a ). R72 and F74 on the convex surfaces of neighbouring Slitrk1 LRR1 domains were found to interact with the backbone of E279 from PTPδ Ig1–3 via hydrophobic interactions and hydrogen bonding, respectively. In addition, R143 on the convex surface of neighbouring Slitrk1 LRR1 domains exhibited weak charge interactions with E230 from PTPδ Ig1–3, which is located in MeB ( Fig. 6b , left). The other packing interaction was mainly mediated by hydrogen bonding between D152 of Slitrk1 LRR1 and R25 of the neighbouring PTPδ Ig1–3 ( Fig. 6b , right). These lateral interaction interfaces, which were distinct from the above-described binding interfaces (that is, the A and B patches; see Fig. 2 ), could potentially contribute to the lateral clustering of LAR-RPTP/Slitrk complexes at the synaptic junction. 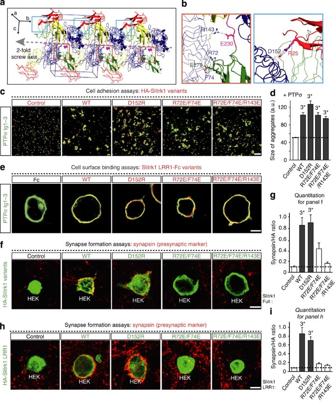Figure 6: Lateral interaction between PTPσ/Slitrk1 complexes for synapse formation. (a) Illustration of the crystal packing interactions of the PTPδ Ig1–3/Slitrk1 LRR1 complex. The colour scheme of PTPδ and Slitrk1 is as described inFig. 2a. The dark blue box represents a unit cell. The lateral interactions introduced by crystal packing are indicated as light blue and orange boxes. The grey arrow represents the two-fold screw axis and the crystallographicbaxis. For clarity, the two alternating PTPδ Ig1–3/Slitrk1 LRR1 complexes are represented as cartoon and ribbon views, respectively. (b) Close-up view of the crystallographic packing interactions shown in the orange box (left) and light blue box (right) ina. The key binding residues mediated by crystal packing are presented. (c,d) Representative images (c) and summary bar graphs (d) for the results of our cell-adhesion assays. One group of L cells co-expressing EGFP and PTPσ Ig1–3 was mixed with a second group of L cells co-expressing DsRed and the indicated Slitrk1 variants. Dark grey bars are significantly different from the control. Scale bar, 100 μm. ‘n’ denotes the total number of cell aggregates from at least three independent experiments (300–1,500 aggregates from 5 to 9 cells); statistical significance indwas assessed using analysis of variance (ANOVA) with Tukey’s test (3*P<0.001). (e) Representative cell surface binding assays. HEK293T cells expressing pDis-PTPs Ig1–3 were incubated with the indicated Slitrk1 LRR1-Fc variants and analysed by immunofluorescence imaging for Slitrk1 LRR1-Fc variants (red) and HA-tagged PTPσ−Ig1–3 (green). Scale bar ,20 μm. Representative images (f,h) and quantification (g,i) of the results from heterologous synapse-formation assays. HEK293T cells transfected with EGFP alone (Control) or the indicated pDis-HA-Slitrk1 mutants (f,g) or pDis-Slitrk1 LRR1 mutants (h,i) were cocultured with hippocampal cultured neurons and immunostained using antibodies against GFP/HA (green) and synapsin (red). ‘n’ in panelsgandidenotes the total number of HEK293T cells analysed. Ing: Control,n=19; WT,n=18; D152R,n=18, R72E/F74E,n=15; and R72E/F74E/R143E,n=19. Ini: Control,n=11; WT,n=14; D152R,n=15, R72E/F74E,n=14; and R72E/F74E/R143E,n=16. Statistical significance (g,i) was assessed using ANOVA with Tukey’s test (3*P<0.001). Scale bar, 30 μm. Figure 6: Lateral interaction between PTPσ/Slitrk1 complexes for synapse formation. ( a ) Illustration of the crystal packing interactions of the PTPδ Ig1–3/Slitrk1 LRR1 complex. The colour scheme of PTPδ and Slitrk1 is as described in Fig. 2a . The dark blue box represents a unit cell. The lateral interactions introduced by crystal packing are indicated as light blue and orange boxes. The grey arrow represents the two-fold screw axis and the crystallographic b axis. For clarity, the two alternating PTPδ Ig1–3/Slitrk1 LRR1 complexes are represented as cartoon and ribbon views, respectively. ( b ) Close-up view of the crystallographic packing interactions shown in the orange box (left) and light blue box (right) in a . The key binding residues mediated by crystal packing are presented. ( c , d ) Representative images ( c ) and summary bar graphs ( d ) for the results of our cell-adhesion assays. One group of L cells co-expressing EGFP and PTPσ Ig1–3 was mixed with a second group of L cells co-expressing DsRed and the indicated Slitrk1 variants. Dark grey bars are significantly different from the control. Scale bar, 100 μm. ‘ n ’ denotes the total number of cell aggregates from at least three independent experiments (300–1,500 aggregates from 5 to 9 cells); statistical significance in d was assessed using analysis of variance (ANOVA) with Tukey’s test ( 3 * P <0.001). ( e ) Representative cell surface binding assays. HEK293T cells expressing pDis-PTPs Ig1–3 were incubated with the indicated Slitrk1 LRR1-Fc variants and analysed by immunofluorescence imaging for Slitrk1 LRR1-Fc variants (red) and HA-tagged PTPσ−Ig1–3 (green). Scale bar ,20 μm. Representative images ( f , h ) and quantification ( g , i ) of the results from heterologous synapse-formation assays. HEK293T cells transfected with EGFP alone (Control) or the indicated pDis-HA-Slitrk1 mutants ( f , g ) or pDis-Slitrk1 LRR1 mutants ( h , i ) were cocultured with hippocampal cultured neurons and immunostained using antibodies against GFP/HA (green) and synapsin (red). ‘ n ’ in panels g and i denotes the total number of HEK293T cells analysed. In g : Control, n =19; WT, n =18; D152R, n =18, R72E/F74E, n =15; and R72E/F74E/R143E, n =19. In i : Control, n =11; WT, n =14; D152R, n =15, R72E/F74E, n =14; and R72E/F74E/R143E, n =16. Statistical significance ( g , i ) was assessed using ANOVA with Tukey’s test ( 3 * P <0.001). Scale bar, 30 μm. Full size image To further investigate the potential biological significance of the lateral interactions observed in crystal packing, we performed cell-adhesion assays, cell surface-binding assays and heterologous synapse-formation assays with mutants designed to abolish the lateral interactions. All of the designed Slitrk1 mutants (D152R, R72E/F74E and R72E/F74E/F143E) appropriately folded and shaped ( Supplementary Fig. 11a,b ), and maintained the binding ability towards PTPσ Ig1–3 ( Fig. 6c–e ; see also Supplementary Fig. 11c for binding-affinity data). Our heterologous synapse-formation assays demonstrated that Slitrk1 R72E/F74E exhibited significantly decreased presynaptic differentiation activity than Slitrk1 WT. Moreover, the addition of the R143E mutation to the Slitrk1 R72E/F74E mutant completely abolished synaptogenic activity. In contrast, the Slitrk1 D152R mutant did not show any alteration of its synaptogenic activity ( Fig. 6f,g ). This conclusion was also confirmed using identical sets of Slitrk1 LRR1 constructs ( Fig. 6h,i ), excluding any possible interaction of these mutant proteins with the Slitrk1 LRR2 domain. Furthermore, to visualize the dynamics of Slitrk1-induced PTPσ clusters on the cell surface, we transiently transfected COS-7 cells with full-length PTPσ-EGFP and examined live cells using time-lapse microscopy. Live-cell imaging revealed that within 5 min after treatment with Slitrk1 LRR1-Fc, PTPσ WT clusters formed at the cell surface, clusters that may represent PTPσ/Slitrk1 signalling cluster ( Fig. 7a,b ; see also Supplementary Movies 1 and 2 ). Strikingly, the addition of Slitrk1 R72E/F74E/F143E-Fc failed to induce the formation of PTPσ clusters ( Fig. 7a,b and Supplementary Movies 1 and 2 ), although this Slitrk1 mutant properly binds to PTPσ ( Fig. 6c,e ). These data strongly support our proposed model that both the binding of Slitrks to LAR-RPTPs and the subsequent lateral clustering of this trans -adhesion complex are crucial for presynaptic differentiation ( Fig. 7c ). 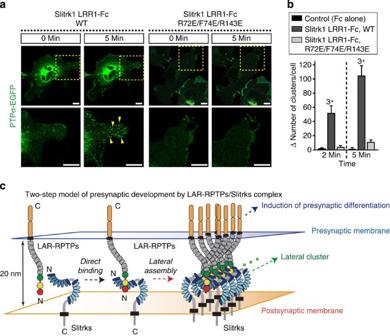Figure 7: Lateral clustering of PTPσ/Slitrk1 complex induced by Slitrk1 binding. (a) Confocal time-lapse images of PTPσ clustering in COS-7 cells induced by addition of Slitrk1 WT-Fc, but not by Slitrk1 F72E/F74E/R143E-Fc (lateral-interaction mutant). Arrowheads indicate the representative clustering events. Scale bar, 20 μm. (b) Quantification of data presented inaat each time point. Error bars represent s.d. from five different cells. Statistical significance was assessed using analysis of variance with Tukey’s test (3*P<0.001). (c) Model of the two-step presynaptic differentiation process mediated by the binding of Slitrks to LAR-RPTPs and subsequent lateral assembly oftrans-synaptic LAR-RPTPs/Slitrk complexes. Figure 7: Lateral clustering of PTPσ/Slitrk1 complex induced by Slitrk1 binding. ( a ) Confocal time-lapse images of PTPσ clustering in COS-7 cells induced by addition of Slitrk1 WT-Fc, but not by Slitrk1 F72E/F74E/R143E-Fc (lateral-interaction mutant). Arrowheads indicate the representative clustering events. Scale bar, 20 μm. ( b ) Quantification of data presented in a at each time point. Error bars represent s.d. from five different cells. Statistical significance was assessed using analysis of variance with Tukey’s test (3* P <0.001). ( c ) Model of the two-step presynaptic differentiation process mediated by the binding of Slitrks to LAR-RPTPs and subsequent lateral assembly of trans -synaptic LAR-RPTPs/Slitrk complexes. Full size image LAR-RPTPs were originally identified as essential elements for early neuron development, but they have recently emerged as synaptic adhesion molecules [2] , [3] . Previous structural studies of LAR-RPTPs focused on the Ig domains [17] , [28] and catalytic phosphatase domains [29] , and provided insights into the arrangement of the Ig domains, the proteoglycan-mediated clustering of the Ig domains and the role of the two tandem phosphatase domains. From a structural perspective, however, we do not yet understand the precise nature of the extracellular interactions between LAR-RPTPs and multiple postsynaptic adhesion molecules. In the present study, we used structural, cell biological and biochemical approaches to address the following major questions left unanswered by previous studies: (1) How do Slitrks specifically bind to LAR-RPTPs? (2) How is the LAR-RPTP/Slitrk interaction regulated by alternative splicing of LAR-RPTPs? (3) How do the specific actions of Slitrks and LAR-RPTPs specify the formation of specific synapse types? To address these rather challenging neuroscience questions, we turned to structural biology in the hopes of identifying the molecular determinants that are crucial for this interaction at an atomic level. This structure–function study yielded four principal observations that address most of the previously unanswered questions regarding the LAR-RPTP/Slitrk synaptic adhesion complex. First, LAR-RPTP Ig1–3 and Slitrk LRR1 constitute the minimal binding regions for their mutual interaction ( Fig. 1 and Supplementary Figs. 1 and 2 ) and are sufficient to mediate their synaptogenic activity ( Fig. 1 and Supplementary Fig. 1 ). Our analysis of the crystal structure of this minimal binding complex revealed that LAR-RPTP Ig2–Ig3 primarily binds to the concave face of Slitrk1 LRR1, forming two crucial binding regions, which we designated the A and B patches ( Fig. 2 ). Extensive functional assays confirmed that a specific subset of residues in the A and B patches are involved in both the LAR-RPTP/Slitrk interaction and synaptogenic activity ( Figs 2 and 3 , and Supplementary Figs 5 and 6 ). Slitrk1 was previously reported to promote excitatory synapse formation through interactions with PTPσ [10] . However, the results of our in vitro biochemical assays as well as synapse-formation assays unequivocally demonstrated that the Slitrk LRR1 domain binds equally well to PTPδ and PTPσ, leading to inhibitory or excitatory presynaptic differentiation, respectively. These findings suggest that the endogenous localizations of various Slitrk and/or LAR-RPTP isoforms, which are temporally and spatially regulated during neuronal development, may determine the specific type of synapse (either excitatory or inhibitory) that is formed in vivo . We also postulate that unique cytoplasmic complexes rather than extracellular protein interactions are critical for driving development of distinct synapse types. Additional studies will be required to elucidate the detailed signalling pathways involved. Second, the MeB splicing insert of LAR-RPTPs was found to regulate the binding to Slitrks ( Fig. 4 ). In cultured neurons and rat brains, the expression level of total and MeB-positive PTPσ gradually decreased during postnatal development ( Fig. 4 ), whereas the total level of Slitrks steadily increased [10] . These data suggest that the interaction of Slitrks with LAR-RPTPs may be involved in initial synaptic specification rather than late synaptic maturation. The significance of alternative splicing in the trans -synaptic adhesion pathway has been extensively explored in the case of the neurexin/neuroligin complex [1] , [30] , [31] . Similar to the case of neurexins, the splicing inserts of LAR-RPTPs alter its binding affinity to various postsynaptic partners, such as TrkC, IL-1RAcP and IL1RAPL1 (refs 2 , 3 ). Further systematic structural analyses of LAR-RPTPs containing various splicing inserts, in complex with diverse postsynaptic adhesion molecules, could unveil general and complex molecular codes for the activation of selective synaptic adhesion pathways. Third, we determined the structural elements that confer the specific binding of LAR-RPTPs to Slitrk LRR1 ( Fig. 5 ). LRR1 and LRR2 are structurally very similar, but our analysis showed that the shape of critical binding pockets and the distribution of specific charged residues in LRR1 impart binding specificity. Although further studies will be required to explore this issue, we propose that Slitrk LRR2 may play yet unidentified roles, such as interacting with other synaptic adhesion molecule. The interaction of Slits with their ligands, the Robos, is comparable to that between LAR-RPTPs and Slitrks, in that both interactions involve the same structural motifs (LRR and Ig domains). In the Slit/Robo interaction, the second LRR domain of Slit binds to the two N-terminal Ig domains of Robo [22] . However, although the Slitrk/LAR-RPTP and Slit/Robo interactions are mediated by common structural motifs, the details of their binding mode appear to be quite different. Specifically, a previous report showed that one face of the β-strand in Robo Ig1 primarily participates in binding to the concave face of the Slit LRR2 (ref. 22 ), whereas we herein report for the first time that the loop connecting Ig2 and Ig3 of LAR-RPTP interacts with the concave face of Slitrk LRR1 ( Fig. 4 and Supplementary Fig. 9c ). These structural comparisons indicate that many protein–protein interactions mediated by the extracellular Ig and LRR domain [32] have evolved to serve divergent functions in the CNS through the specific binding of distinct partners. Fourth, we found that the lateral assembly between adjacent PTPδ Ig1–3/Slitrk1 complexes, which was observed in our crystal-packing lattice, was critical for the synaptogenic activity of Slitrks. Strikingly, Slitrk1 point mutants designed to abolish these crystal-packing interactions impaired presynaptic differentiation in our heterologous synapse-formation assays, but did not affect the primary PTPδ/Slitrk1 binding ( Fig. 6 ), suggesting that the binding of Slitrks to their presynaptic ligands is not sufficient to induce presynaptic differentiation. Although we failed to observe multimeric PTPδ/Slitrk1 complexes in solution, the demonstration of Slitrk1-mediated clustering of PTPσ/Slitrk1 complexes on the cell membrane by time-lapse microscopy ( Fig. 7 ) strongly suggests that the lateral assembly of these trans -synaptic adhesion complexes is physiologically relevant and may be crucial for efficient propagation of downstream signals required for proper presynaptic differentiation. Other postsynaptic partners of LAR-RPTPs could also synergistically and/or cooperatively form a variety of trans/cis -synaptic adhesion networks. A previous study has suggested that the catalytic activity of LAR-RPTP most probably undergoes negative regulation via dimerization (ligand-induced or otherwise) [33] . Moreover, a prior study showed that heparan sulfate proteoglycans induce the clustering of PTPσ, thus facilitating neuronal extension by unevenly distributing phosphatase activity at the cell surface [17] . Although additional studies are needed to further clarify the Slitrk-binding-induced conformational changes and/or oligomerization of LAR-RPTPs, the higher-order architecture initiated by the binding of Slitrks to LAR-RPTPs could be a key event in the bidirectional neuronal signal transduction. This could then lead to further synaptogenic processes, as has been proposed for the higher-order architecture of neurexin/neuroligin, cadherins, SynCAM1 and Eph/Ephrin [23] , [24] , [25] , [26] , [27] , [34] , [35] . In conclusion, we herein used structural and functional studies to probe the significance of the interaction between LAR-RPTPs and Slitrks during synapse formation, and provide a molecular basis for the regulation of this interaction by alternative splicing (particularly that involving the splicing insert, MeB). Moreover, we dissected the process of Slitrk-induced presynaptic differentiation into two molecular steps as follows: (1) the direct binding of postsynaptic Slitrks to presynaptic LAR-RPTPs and (2) lateral clustering mediated by the initially formed monomeric LAR-RPTP/Slitrk trans -synaptic complexes ( Fig. 7c ). These rearrangements of the extracellular architecture are likely to change the catalytic activity of the intracellular phosphatase in LAR-RPTPs, thereby inducing the recruitment of nascent presynaptic machineries. Future studies should examine whether multimeric LAR-RPTPs are catalytically active, how their multivalent binding with multiple postsynaptic ligands can be modulated and how the activations of downstream signalling pathways are specified. Construction of expression vectors All of the constructs used in this study are summarized in Supplementary Table 1 . MeA (ETFESTPIR for PTPσ; ESIGGTPIR for PTPδ; GGSPIR for LAR) and/or MeB (ELRE for both PTPσ and PTPδ; DQRE for LAR) were introduced into the pDis-PTPσ Ig1–3 (MeA−, MeB−) and pDis-PTPδ Ig1–3 (MeA−, MeB−) construct to yield splice variants containing the combination of MeA and MeB splicing inserts. We additionally generated pDis-PTPσ Ig1–3 ΔEVR, in which three amino acids (E239, V240 and R241) were deleted from pDis-PTPσ Ig1–3. Recombinant expression and purification The ectodomain fragments of human PTPδ (aa 21E–322L) and PTPσ (aa 30E–331L), which had been cloned into the BamHI and XbaI sites of the pAcGP67 vector (BD Biosciences), were fused to the protein A gene derived from pEZZ18 (GE Healthcare Life Sciences). The ectodomain fragment of Slitrk1 LRR1 (aa 20T–264K) or Slitrk1 LRR2 (aa 337N–580Q), which had been cloned into the BamHI and NotI sites of the pAcGP67 vector (BD Biosciences), were fused to the Fc domain of the human IgG gene ( Supplementary Table 1 ). A thrombin cleavage site (LVPRGS) was introduced between the target and tagging genes. PTP ectodomain fragments (PTPδ Ig1–3 and PTPσ Ig1–3) and Slitrk1 ectodomain fragments (Slitrk1 LRR1, Slitrk1 LRR2 and Slitrk1 Full) were expressed in High Five insect cells (Invitrogen). High Five cells transfected with the corresponding P4 baculovirus were incubated for 3 days and then pelleted by centrifugation. The supernatants containing secreted proteins were pooled and loaded onto IgG Sepharose columns (GE Healthcare Life Sciences) for the purification of the protein A-fused PTP ectodomain fragment, or protein A sepharose columns (GE Healthcare Life Sciences) for purification of the Slitrk1-Fc (Slitrk1 LRR1-Fc, Slitrk1 LRR2-Fc and Slitrk1 Full-Fc). The affinity resin was washed (50 mM Tris-Cl, pH 8.0, and 200 mM NaCl) and then treated with thrombin (0.5% (v/v) in 20 mM Tris-Cl, pH 8.0, and 200 mM NaCl) at 4 °C overnight to remove the C-terminal protein A or Fc tags. The buffer was changed to 20 mM MES, pH 6.5, and cleaved proteins were loaded onto a cation-exchange HiTrap SP column (GE Healthcare Life Sciences) and eluted with a 0–1 M NaCl gradient. Fractions containing recombinant proteins were further purified by gel-filtration chromatography on a Superdex 200 column (GE Healthcare Life Sciences) equilibrated with 20 mM Tris-Cl, pH 8.0, and 200 mM NaCl, and then concentrated for crystallization. The PTPδ Ig1–3/Slitrk1 LRR1 complex was produced by mixing purified Slitrk1 LRR1 (11 μM in 840 μl) with PTPδ Ig1–3 (63 μM in 120 μl) and incubating the mixture for 3 h at 4 °C. Thereafter, unbound Slitrk1 LRR1 was excluded by gel filtration chromatography (buffer: 20 mM Tris-Cl, pH 8.0, and 200 mM NaCl). Fractions containing the PTPδ Ig1–3/Slitrk1 LRR1 complex, which were forward shifted in the chromatographic profile, were pooled and further concentrated to 4 mg ml −1 for crystallization. Pull-down assays Slitrk1 LRR1-Fc, Slitrk1 LRR2-Fc, Slitrk1 Full-Fc and Fc alone (20 μg) were individually incubated with 30 μl protein A sepharose (50% slurry; GE Healthcare Life Sciences) at room temperature for 1 h. The beads were washed three times with PBS and then incubated with 40 μg of PTPσ Ig1–3 or PTPδ Ig1–3 at room temperature for 1 h. The unbound proteins were removed by washing with PBS and the resin-bound proteins were solubilized by boiling in 5 × SDS–PAGE sample buffer and analysed by 10% SDS–PAGE. Cell-adhesion assays Cell-adhesion assays were performed using L cells as described previously [36] . Briefly, two groups of L cells plated in six-well plates were transfected individually with the expression vectors, as indicated. After 48 h, the cells were trypsinized and resuspended in DMEM and the two groups of L cells were mixed and rotated at room temperature to allow the cells to aggregate. The extent of cell aggregation was measured after 2 h; aliquots were spotted onto four-well culture slides and imaged by confocal microscopy. For quantification of the number of cells per cluster, cell clusters were defined as cell aggregates that contained four or more cells and included at least one green (EGFP) and one red (DsRed) cell. Frames with no detectable cell clusters were counted as zero. The data are presented as means±s.e.m. ( n =10–15 fields from at least three independent experiments). Heterologous synapse-formation assays Heterologous synapse-formation assays were performed using HEK293T cells, as described previously [37] . Briefly, for the experiments shown in Fig. 3d,e , HEK293T cells were transfected with EGFP (negative control), pCMV5-Slitrk1-mVenus WT, or the various pCMV5-Slitrk1-mVenus point mutants (described in the ‘List of point mutant plasmids generated for this study’; see also Supplementary Table 3 ) using FuGene-6 (Roche). For the experiments shown in Supplementary Fig. 6c , HEK293T cells were transfected with EGFP, pDis-HA-Slitrk1 WT, or the various pDis-HA-Slitrk1 point mutants. After 48 h, HEK293T cells transfected with the indicated expression vectors, were trypsinized, seeded onto hippocampal neuron cultures at DIV9, further cocultured for 72 h and then (at DIV12) double-immunostained with antibodies against GFP and synapsin I, VGLUT1 or VGAT [36] . All images were acquired with a confocal microscope (LSM510, Zeiss). For quantification, the contours of transfected HEK293T cells were chosen as the region of interest. The fluorescence intensity of immunoreactive puncta were normalized with respect to each HEK293T cell area and then quantified for both red and green channels using the MetaMorph Software (Molecular Devices). The data are given as means±s.e.m. ( n =18–24 HEK293T cells; 3 * P <0.001). Affinity measurement by solid-phase protein-binding assays The affinity of Slitrk1 for LAR-RPTPs was determined using a solid-phase protein-binding assay. Each variant (PTPδ Ig1–3, PTPσ Ig1–3) in PBS was immobilized on Maxi-Sorp 96-well plates (NUNC; 1 μg per well) by incubating for 2 h at 37 °C. Nonspecific binding was blocked by incubating wells with 1% skim milk. After blocking, Fc-fused Slitrk1 LRR1, LRR2 or LRR1+LRR2 protein at different concentrations (0.05, 0.1, 0.2, 0.3, 0.4, 0.5, 0.75, 1 and 2 μM) in 1% skim milk was added and plates were incubated for 2 h at 37 °C. After washing three times with PBS, horseradish peroxidase-conjugated anti-human Fc antibody (1:10,000; Sigma) was added. Immunoreactive proteins were detected by developing with TMB substrate (KPL) for 5 min. Thereafter, the reaction was quenched by the addition of 1 M HCl and absorbance was measured at 450 nm using a Model 680 microplate reader (Bio-Rad). Absorbance values were plotted against Slitrk1 concentration and K D values were determined by fitting the curves to a one-site binding model by nonlinear regression using GraphPad Prism 6. Crystallization and structural determination Crystals of PTPδ Ig1–3/Slitrk1 LRR1 complex were grown for 1 week using the hanging-drop vapour-diffusion method, in which 1 μl of protein complex (4 mg ml −1 ) was mixed with 1 μl of crystallization buffer containing 100 mM Tris-Cl, pH 8.5, 200 mM ammonium sulfate and 20% PEG3350 (v/v). Crystals of the PTPδ Ig1–3/Slitrk1 LRR1 complex belonged to space group P2 1 and had the following unit cell constants: a =77.28 Å, b =60.37 Å, c =84.14 Å, α =90.00°, β =102.14° and γ =90.00°. For data collection at 100 K, crystals were transferred to a cryoprotective solution containing 100 mM Tris-Cl, pH 8.5, 200 mM ammonium sulfate, 23% PEG3350 (v/v) and 30% glycerol (v/v), and shock frozen in liquid nitrogen. Crystals of Slitrk1 LRR2 were grown for 1 week using the hanging-drop vapour-diffusion method, in which 1 μl of protein solution (1 mg ml −1 ) was mixed with 1 μl of crystallization buffer containing 100 mM Na-citrate, pH 5.5, 16% isopropanol and 12% PEG4000 (v/v). Slitrk1 LRR2 protein crystals belonged to space group P6 1 22 and had the following unit cell constants: a =69.70 Å, b =69.70 Å, c =410.20 Å, α =90.00°, β =90.00° and γ =120.00°. For data collection at 100 K, crystals were transferred to a cryoprotective solution containing 100 mM Na-citrate, pH 5.5, 16% isopropanol, 15% PEG4000 (v/v) and 30% glycerol (v/v), and shock frozen in liquid nitrogen. Diffraction data for crystals of Slitrk1 LRR2 and the PTPδ Ig1–3/Slitrk1 LRR1 complex were collected at beamline 5.0.2 (Advanced Light Source) and 7A (Pohang Accelerator Laboratory), respectively. The initial phases were calculated by the molecular replacement technique using the PHASER programme [38] . The structure of variable lymphocyte receptor A (PDB ID: 3M18) [20] , which has a six LRR motif, was used as a search probe for the structure determination of Slitrk1 LRR2. The refined Slitrk1 LRR2 structure and the first Ig domain of PTPδ (PDB ID: 2YD6) [17] were used as search models to determine the structure of the PTPδ Ig1–3/Slitrk1 LRR1 complex, using the molecular replacement technique. The atomic models were refined by iterative rounds of model building performed using the Coot programme [39] and refinements with CNS [40] , Refmac [41] and PHENIX [42] programmes. The statistics for our data collection and refinements are summarized in Table 1 . The quality of each model was checked using the PROCHECK analysis tool [43] . Ramachandran plot analysis of the PTPδ Ig1–3/Slitrk1 LRR1 complex structure showed that 95.5%, 4.3% and 0.2% of residues were located in favoured regions, allowed regions and outlier regions, respectively. The percentages of residues in the Ramachandran favoured regions, allowed regions and outlier regions for the Slitrk1 LRR2 crystal structure were 95.2%, 4.8% and 0.0%, respectively. Antibodies The following primary antibodies were used in this study: anti-synapsin I (1 μg ml −1 , rabbit polyclonal; Millipore), anti-VGLUT1 (1 μg ml −1 , guinea pig polyclonal; Millipore), anti-VGAT (1 μg ml −1 , rabbit polyclonal; Synaptic Systems), anti-HA (1 μg ml −1 , mouse monoclonal, clone HA-7; Covance) and anti-EGFP (1 μg ml −1 , goat polyclonal; Rockland). The following secondary antibodies were used: Cy3-conjugated anti-rabbit, Cy3-conjugated anti-guinea (1 μg ml −1 ), fluorescein isothiocyanate (FITC)-conjugated anti-goat (1 μg ml −1 ), FITC-conjugated anti-mouse (1 μg ml −1 ) and Cy5-conjugated anti-mouse (1 μg ml −1 ) (all from Jackson ImmunoResearch). Site-directed mutagenesis The Slitrk1 and PTPσ point mutants, described in Supplementary Table 3 were generated with a QuickChange site-directed mutagenesis kit (Stratagene) and verified by DNA sequencing. The PTPσ and Slitrk1 residues are numbered with respect to the human PTPσ (AAX50299.1) and Slitrk1 (NP_443142.1) sequence, respectively, which was previously described [5] , [12] . Cell surface-binding assays Slitrk1 LRR1-Fc (WT and point mutants; Supplementary Tables 1 and 3 ) were produced from High Five insect cells as described for the proteins that were used for crystallization. Recombinant Slitrk1 LRR1-Fc variants were purified with protein A-sepharose beads (GE Healthcare Life Sciences). Instead of the thrombin cleavage step used for the purification of the crystallization proteins, the Slitrk1 LRR1-Fc variants were eluted with 100 mM glycine, pH 3.0, and immediately neutralized with 1 M Tris-Cl, pH 8.0. Transfected HEK293T cells expressing pDis-PTPσ Ig1–3 point mutants (Y233S, R235A, R238A, R235D/R238D, S248A or S248A/R295A) or EGFP (negative control) were incubated with 0.2 μM Fc or Slitrk1 LRR1-Fc WT, as indicated in Fig. 3b . Transfected HEK293T cells expressing pDis-PTPσ Ig1–3 WT or DsRed (negative control) were incubated with 0.2 μM Fc, Slitrk1 LRR1-Fc WT or Slitrk1 LRR1-Fc mutants (Y134R, 134W, 157A, I160W, N162R, D163R/D211R or Q248A) as indicated in Fig. 3c . Images were acquired using a confocal microscope (LSM510; Zeiss). Primary neuron culture and immunocytochemistry Rat hippocampal cultures were prepared from E18 (embryonic day 18) embryos [44] . Briefly, rat hippocampus at E18 were dissected out, trypsinized and triturated to single-cell suspension. These cells were cultured in neurobasal medium (Life Technologies). For immunocytochemistry, cultured neurons were fixed with 4% paraformaldehyde/4% sucrose for 10 min at room temperature, permeabilized with 0.2% Triton X-100 in PBS for 5 min at 4 °C, blocked with 3% horse serum/0.1% crystalline grade BSA in PBS for 30 min at room temperature and sequentially incubated with the indicated primary and secondary antibodies in blocking solution for 1 h at room temperature. Transfected cells were randomly chosen and acquired using a confocal microscope (LSM510; Zeiss) with a × 63 objective lens; all image settings were kept constant. Z -stack images obtained by confocal microscopy were converted to maximal projections and analysed for intensity at the presynaptic terminals using the MetaMorph software (Molecular Devices). All images were separated by their colour channels (red and green), and red-coloured images were transformed into grey-scale images using Photoshop (Adobe). All analyses were performed in a blinded manner. Biotinylation assays in HEK293T cells HEK293T cells expressing pCMV5-Slitrk1-mVenus WT or its point mutants were rinsed with PBS containing 1 mM MgCl 2 and 1 mM CaCl 2 , and then incubated with 1.0 mg ml −1 Sulfo-NHS-LC-biotin (Thermo Scientific) in PBS for 30 min at 4 °C. The cells were rinsed in 100 mM glycine in PBS to quench any unbound biotin, and then extracted in lysis buffer (1% Triton X-100, 0.1% SDS) containing a complete protease inhibitor cocktail (Roche). Biotinylated proteins were purified using NeutrAvidin agarose (Pierce), separated by SDS–PAGE and analysed by western blotting with anti-EGFP antibodies. Surface labelling assays in HEK293T cells Transfected HEK293T cells expressing haemagglutinin-tagged Slitrk1 WT or the indicated Slitrk1 mutants were incubated overnight at 4 °C with 1 μg ml −1 mouse anti-HA antibody in DMEM containing 20 mM HEPES, pH 7.4, and 0.1% BSA. The cells were then washed with PBS, fixed with 4% paraformaldehyde for 10 min on ice, blocked with 3% skim milk in PBS for 30 min at room temperature and incubated with anti-mouse Cy3 antibodies (1:500 in blocking solution) for 1 h at room temperature. Cells are then permeabilized with 0.2% Triton X-100 in PBS for 5 min on ice, washed and incubated with rabbit anti-HA antibody in DMEM containing 20 mM HEPES, pH 7.4, and 0.1% BSA for 1 h at room temperature to label intracellularly endocytosed Slitrk1 proteins. Immunoreactive proteins were detected by incubation with FITC-conjugated anti-rabbit secondary antibodies (1:150 in blocking solution). All experiments were repeated three times. KD PTPσ and rescue in hippocampal neurons Recombinant lentiviruses were produced by triply transfecting HEK293T cells with three plasmids—lentiviral transfer vectors (L-309 alone, L-309 PTPσ-KD, L-313 PTPσ MeA−/MeB+, or L-313 PTPσ MeA−/MeB−), psPAX and pMD2G—using FuGene-6 (Roche) [10] , [45] . The psPAX and pMD2G plasmids encode the elements essential for packaging viral particles. HEK293T cell supernatants were harvested 48 h post transfection and purified [46] . Hippocampal neurons infected at DIV3 with control lentiviruses (sh-Control) or shRNA targeting PTPσ (sh-PTPσ) or co-infected with lentiviruses expressing PTPσ shRNA plus the human shRNA-resistant PTPσ splice variant with an MeB insert (+PTPσ MeB+), or PTPσ shRNA plus the human shRNA-resistant PTPσ splice variant without an MeB insert (+PTPσ MeB−). The infected neurons were then cocultured for 2 days with HEK293T cells transfected with EGFP alone (Control) or HA-Slitrk1 (Slitrk1), and stained with antibodies against HA or EGFP (green) and VGLUT1 (red). KD efficacy was measured using qRT–PCR with primer set (5′- GAA CCG ATA CGC CAA TGT CA -3′: forward and 5′- TCA CTA CCC ATG ATG CCT TCT AAA -3′: reverse). qRT–PCR in cultured hippocampal neurons and rat brains Rat cultured hippocampal neurons plated on a 12-well plate were homogenized at DIV5, DIV10, DIV15 and DIV20 in TRIzol Reagent (Invitrogen) and total RNA was extracted according to the manufacturer’s protocol. The corresponding complementary DNA was prepared from the total RNA by random priming using a cDNA synthesis kit (Takara Bio). Quantitative real-time PCR was performed using a CFX96 Real-Time PCR system (BioRad) and SYBR green reagents (Takara Bio). Primer sequences were designed to detect MeB-containing splice variants of rat PTPσ or rat PTPδ. The ubiquitously expressed mRNA, glyceraldehyde-3-phosphate dehydrogenase, was detected as an endogenous control. RT–PCR values are presented as the ratio of the signal obtained from the specific PTPσ or PTPδ splice variant versus that from total PTPσ or PTPδ, respectively. The following primer pairs were used: PTPσ (MeB+), 5′- GAG AGC TTC GAG AAG T -3′ (forward) and 5′- CTC TGC CCC CTG CAT CCA CTT -3′ (reverse); PTPδ (MeB+), 5′- TTC AGG TGT CAG ATC TTC TGC -3′ (forward) and 5′- CTC GGC CCC CTG CAT CCA CTT -3′ (reverse); PTPσ (total), 5′- GAG AGC TTC GAG AAG T -3′ (forward) and 5′- CTC TGC CCC CTG CAT CCA CTT -3′ (reverse); PTPδ (total), 5′- TTC AGG TGT CAG ATC TTC TGC -3′ (forward) and 5′- CTC GGC CCC CTG CAT CCA CTT -3′ (reverse); glyceraldehyde-3-phosphate dehydrogenase, 5′- TGA TGA CAT CAA GAA GGT GAA G -3′ (forward) and 5′- TCC TTG GAG GCC ATG TAG GCC AT -3′ (reverse). Total RNA was isolated from P1, P14 or P28 rat brains using the TRIzol reagent and was used for cDNA synthesis. To examine the role of network activity in regulating the expressions of PTPσ, we treated cultured hippocampal neurons at DIV5–10 with 20 μM NBQX, 50 μM D-APV, 25 μM 4-aminopyridine or 50 μM bicuculline for 72 h, or with 2 μM tetrodotoxin (all from Tocris Bioscience) for 2 h. Negative-stained TEM analysis and image processing Slitrk1 Full (240 nM) was applied to a glow-discharged carbon-coated 400 mesh copper grid (Electron Microscopy Science), which was then stained with 0.75% uranyl formate solution (Electron Microscopy Science) [47] . Images were acquired using a Tecnai T12 Bio-TWIN transmission electron microscope equipped with an FEI Eagle 4 × 4 K charge-coupled device camera and operating at 120 kV. Particles ( n =1,403) for Slitrk1 Full were manually selected from 100 micrographs using the EMAN2 boxer programme [48] . The particles were subjected to three rounds of multivariate statistical analysis classification and multi-reference alignment using IMAGIC [49] . Next, the 1,403 particles were grouped into six classes (~230 particles per class). The class averages were sorted by the overall quality based on Representation quality and Variance/Member analysed by IMAGIC. For the two-dimensional class average of Slitrk1 LRR1 WT or mutants, ~600 particles were selected from 30 micrographs and image processing were performed similarly as image processing for Slitrk1 Full. Live-cell imaging COS-7 cells were cultured and transfected with a PTPσ-EGFP construct using Lipofectamine LTX (Invitrogen). After 12–18 h, the medium was replaced with DPBS containing glucose (Invitrogen). Cells were treated with 10 μg ml −1 of recombinant WT or lateral-interaction mutant (R72E/F74E/F143E) Slitrk1 LRR1-Fc protein and imaged every 30 s for 7 min with a confocal microscope (Nikon A1) at × 60 magnification. PTPσ/Slitrk1 complex clusters were detected by monitoring the fluorescence of EGFP, C-terminally fused to PTPσ. MetaMorph Software (Molecular Devices) was used to assemble movies and quantify Slitrk1-mediated surface clusters. For purposes of quantification, clusters were defined as discrete puncta of fluorescence that satisfied criteria of size (>5 pixel) and circularity (0.1~1.0) [50] . Circular dichroism The secondary structures of purified SlitrK1 and its mutants (R72E/F74E and R72E/F74E/R143E) are monitored by circular dichroism (CD) at 20 °C in 1 mm cell. The concentrations of SlitrK1 WT and its mutants (R72E/F74E and R72E/F74E/R143E) for measurement are 53.9, 49.3 and 55.8 μM, respectively. CD spectra were recorded using a Jasco J-815 CD spectrometer between 190 and 230 nm at 1-nm intervals averaged over 1 s. The molar ellipticity ([ θ ]molar) is calculated by equation described below. where, θ obs is the observed value of CD, d is distance of measuring cell and m is molar concentration of the protein. Statistics All data are expressed as means±s.e.m. All experiments were performed on at least three independent cultures and were evaluated statistically using the Student’s t -test or the analysis of variance Tukey test, with the number of experiments used as the basis for ‘n’ (* P <0.05, 2 * P <0.01; 3 * P <0.001). How to cite this article: Um, J. W. et al . Structural basis for LAR-RPTP/Slitrk complex-mediated synaptic adhesion. Nat. Commun. 5:5423 doi: 10.1038/ncomms6423 (2014). Accession codes: Atomic coordinates and structural features have been deposited in the Protein Data Bank under accession codes 4RCA (PTPδ Ig1–3/Slitrk1 LRR1 complex) and 4RCW (Slitrk1 LRR2).